Complex self-assembly of pyrimido[4,5-d]pyrimidine nucleoside supramolecular structures Supramolecular self-assembly is not only one of the chemical roots of biological structure but is also drawing attention in different industrial fields. Here we study the mechanism of the formation of a complex flower-shaped supramolecular structure of pyrimido[4,5- d ]pyrimidine nucleosides by dynamic light scattering, scanning electron microscopy, differential scanning calorimetry, nuclear magnetic resonance and X-ray analysis. Upon removing the hydroxyl group of sugars, different flower-shaped superstructures can be produced. These works demonstrate that complex self-assembly can indeed be attained through hierarchical non-covalent interactions of single molecules. Furthermore, chimerical structures built from molecular recognition by these monomers indicate their potential in other fields if combined with other chemical entities. Biological structures developed by living organisms have their chemical roots in molecular (covalent) and supramolecular (non-covalent) morphogenesis and are currently at the frontiers of physics, chemistry, biology and other disciplines with high hopes to generate novel entities and properties [1] , [2] , [3] , [4] , [5] , [6] . Some micro- and nano-structures with plant-like morphologies have been reported [7] , [8] , [9] , [10] , [11] , [12] , [13] . Recently, highly branched flower-shaped structures have attracted attention due to their potential in the fields of magnetic materials, catalysis, optoelectronic devices, solar cells and medicine [14] , [15] , [16] , [17] , [18] , [19] . Previously, the flower-shaped structures were mainly synthesized by covalent inorganic species. Later, a fullerene derivative was reported to be the first flower-shaped organic supramolecular micro-structure synthesized through the combination of the π–π interaction of C 60 and the van der Waals interaction of aliphatic side chains [20] , [21] . Certain flower-shaped assemblies of benzothiophene derivatives also showed superhydrophobic properties due to this special morphology [22] , [23] . Very recently, a protein-inorganic hybrid nanoflower has been reported with the advantages of enhancing enzymatic activity and stability [24] . Another type of life’s central molecules, nucleic acids (DNA/RNA), have been exploited at polymeric level, with advantages of high-fidelity molecular recognitions and programmable synthesis, to assemble nanowires, lattices and 3D octahedron superstructures, and have found many applications (not only as genetic materials) in nanotechnology [25] , [26] , [27] , [28] , [29] , [30] , [31] . Nucleosides, with specific base–base interactions, have also been used to construct certain supramolecular structures at monomeric level, such as G-quartets, columnar nanotubes and nanoparticles [32] , [33] , [34] . However, using them to construct structures with complex shapes is a relatively unexplored area. Varieties of nucleobase moieties other than canonical purines and pyrimidines have been developed to construct novel superstructures through diverse base pair patterns [35] , [36] , [37] , [38] , [39] . For instance, the Janus-type guanine–cytosine base derivatives have been reported to form rosette nanotubes (RNTs) [35] , [38] . Inspired by these works, we designed and synthesized a series of Janus-type pyrimido[4,5- d ]pyrimidine nucleosides combining all of the four chemical letters of the genetic alphabet, tridentate guanine–cytosine and bidentate adenine–thymine (uracil) nucleosides [40] , [41] . In the attempt to build nanostructures with these nucleosides through their self-complementary two-faced base pair motifs, serendipitously and excitingly, we found that compound 1 (J-AT) can form a complicated and aesthetically appealing flower-shaped superstructure in solution, which was the first report of flower-shaped morphology formed by nucleoside derivatives [42] , [43] . Regrettably, there was no insight into the formation process and finer molecular architectures of these assemblies obtained at that time. Herein we reveal its formation mechanism by time-elapsed SEM, DLS, DSC and VT-NMR. The inner atomic-level molecular interactions are revealed by single-crystal X-ray analysis. In addition, different flower-shaped species are constructed and the recognition property of this flower-shaped structure is investigated. Previously, due to directional restrictions, H-bonds mainly directed the formation of spatially regular micro- or nanostructures in the case of conformational rigid small molecules. In the current case, because of the intrinsic three-dimensional structure and flexible conformation of nucleosides, complex flower-shaped supramolecular morphologies have been constructed and it epitomizes that the reproducing and tailoring of complex structures through hierarchical non-covalent interactions with relatively singular molecules are achievable only by fine tuning the structural parameters. Stability of the flower-shaped superstructure Upon construction of supramolecular structures with pyrimido[4,5- d ]pyrimidine nucleosides, we found that compound 1 (J-AT) formed flower-shaped superstructures with uniform diameters of ~40 μm as observed by SEM and DLS ( Fig. 1 , Supplementary Fig. 1 ), which is drastically different from the microsphere-shaped structures formed by the 2′-deoxyribonucleoside 2 under the exact same conditions. Such flower-shaped superstructures were stable up to 60 days, and no pronounced changes in sizes and morphologies were found during the whole period, indicating that neither collapse nor aggregation occurred. The influence of pH on the stability of the flower-shaped superstructure was checked ( Supplementary Fig. 2 ). The microflower was stable over a wide pH, ranging from 3 to 11. Below pH 3 microspheres and smooth membranous structure were produced, and above pH 11 fibrous structures and nano-particles were produced. 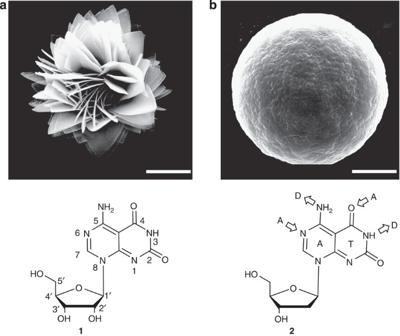Figure 1: SEM images and molecular structures of compounds 1 and 2. (a) Flower-shaped superstructure self-assembled by1in water (0.2 mg ml−1) and its molecular structure with the systematic numbering. (b) Microsphere superstructure self-assembled by2in water (0.2 mg ml−1) and its molecular structure showing the two-faced hydrogen bond acceptor–donor motif of adenine and thymine: the arrows ofAat A represent the hydrogen acceptors and the arrows atDrepresent the hydrogen donors. Scale bars, (a) 10 μm; (b) 5 μm. Figure 1: SEM images and molecular structures of compounds 1 and 2. ( a ) Flower-shaped superstructure self-assembled by 1 in water (0.2 mg ml −1 ) and its molecular structure with the systematic numbering. ( b ) Microsphere superstructure self-assembled by 2 in water (0.2 mg ml −1 ) and its molecular structure showing the two-faced hydrogen bond acceptor–donor motif of adenine and thymine: the arrows of A at A represent the hydrogen acceptors and the arrows at D represent the hydrogen donors. Scale bars, ( a ) 10 μm; ( b ) 5 μm. Full size image Like other self-assembly systems, the formation of such flower-shaped structure was concentration dependent ( Supplementary Fig. 3 ). When the concentrations of compound 1 were above 0.1 mg ml −1 up to the saturated 0.5 mg ml −1 , the flower-shaped superstructures were observed. However, at concentrations below 0.1 mg ml −1 only microspheres were observed, which could be taken as the threshold of the phase transition between two states just like the critical micelle concentration (CMC) is needed for the surfactant to assemble a micelle [44] . The formation process of the microspheres in solution at lower concentrations was monitored by temperature-variant DLS measurements and the dependence of the distribution of hydrodynamic radius of the particles on temperatures indicated that the microspheres observed under SEM were not the result of solvent evaporation ( Supplementary Fig. 4 ). Formation process of the flower-shaped superstructure To investigate the formation mechanism of the flower-shaped superstructure, time-elapsing experiments were carried out. From the samples taken at different time intervals between 0 min and 14 h, it can be seen that the flower-shaped superstructure was growing from the microspherical structure ( Fig. 2a–g ). Only complete microflowers were observed from all the samples taken after 14 h ( Fig. 2h,i ). These phenomena suggested that the formation of the microflowers also happened in the solution, not as a mere result of surface deposition; otherwise, the same shapes should be observed at different time intervals. The time-dependent SEM images also suggested the following mechanism for the formation of the flower-shaped superstructure. In the first stage a spherical nucleation was formed (indicated by low-concentration DLS and SEM); in the second stage the ‘petals’ radially protruded from the surface and grew into the final fully shaped flower, with the gradual fading of the spherical ‘bud’ ( Fig. 2f ). 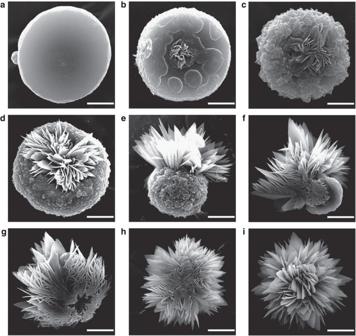Figure 2: SEM images showing the formation process of the flower-shaped superstructure. (a–g) Intermediates of incomplete microflowers were observed within 14 h, which was in a quite similar manner mimicking the natural flowers blooming from buds. (h,i) only the fully unfolded microflowers were observed after 14 h (h, backside;i, frontside). Scale bars, (a–c) 5 μm; (d–i) 10 μm. Figure 2: SEM images showing the formation process of the flower-shaped superstructure. ( a – g ) Intermediates of incomplete microflowers were observed within 14 h, which was in a quite similar manner mimicking the natural flowers blooming from buds. ( h , i ) only the fully unfolded microflowers were observed after 14 h ( h , backside; i , frontside). Scale bars, ( a – c ) 5 μm; ( d – i ) 10 μm. Full size image The energetics of this phase transition was also characterized by DSC, in order to determine the thermodynamic parameters of non-covalent interactions. The overall thermal effects detected were very weak due to the relatively low concentration of the solution; thus, a high-precision microcalorimeter was used. The DSC melting profile of compound 1 (0.4 mg ml −1 ) in water ( Supplementary Fig. 5 ) also indicated two-phase transitions in accordance with the visual evidences of SEM. The thermodynamic information was obtained as: ( T m−1 =50.8 °C, Δ H cal−1 =−1,259.4 kJ mol −1 , Δ G 25−1 =−132.2 kJ mol −1 and T m−2 =63.6 °C, Δ H cal−2 =−93.3 kJ mol −1 , Δ G 25−2 =−79.7 kJ mol −1 ). The Δ G 25 °C of the low-temperature transition is much larger than that of the high-temperature transition. To investigate the non-covalent interactions that direct the formation of such flower-shaped superstructure, the hydrogen bonds were first investigated by the variable-temperature 1 H NMR (VT-NMR) in DMSO ( d 6 ). For the base moiety, the chemical shift of N11HA involved in the intramolecular H-bond remained unchanged, but the chemical shifts of N11HB and N3H involved in intermolecular H-bonds displayed significant changes upon varying temperature ( Supplementary Fig. 6 ). For the sugar residue, the H-bonds resulting from hydroxyl groups in solution state were also observed: for instance, the chemical shift for 2′-OH of the sugar moiety moving from δ 5.33 (363 K) to δ 5.58 p.p.m. (293 K), with Δ δ =0.25 p.p.m. ( Supplementary Fig. 7 ). It is worthwhile mentioning that H-bonds from both base moiety and sugar residues displayed biphasic melting transitions as well (the melting curves of N11HB and 2′-OH are given as examples in Supplementary Fig. 8 ) and the reversibility was confirmed by the overlapping of the VT-NMR melting curves between heating and cooling processes. As the difference of molecular structure between compound 1 and 2 lies only on the 2′-OH group, we supposed that the 2′-OH group plays a key role in the direction of the formation of the flower-shaped supramolecular structures. However, the specific connectivities of these groups could not be solved by this method. To decipher the inner workings of this superstructure at atomic level, we therefore tried to get the single crystal of compound 1 from water for X-ray analysis. Single-crystal structure of compound 1 The preparation of the single crystal was carried out in a much slower process by cooling the saturated aqueous solution of 1 from 100 to 30 °C in steps of 0.5 °C/h in an incubator. Colourless needle single crystals suitable for X-ray diffraction were obtained in 1 week. This was the very first example of a crystalline free pyrimido[4,5- d ]pyrimidine nucleoside and unusual structural features were found. Inspection of the single crystal of 1 disclosed the co-existence of two conformers in equal amounts ( Supplementary Data 1 ). These two conformers, A ( Fig. 3a ) and B ( Fig. 3b ), were different in all the three interacted fundamental structure parameters for nucleosides. We used the torsion angle χ (O4′-C1′-N8-C9) to indicate the rotational position of the nucleobase relative to the sugar ring ( syn/anti conformation) for pyrimido[4,5- d ]pyrimidine nucleosides. The torsion angles χ of conformers A and B were measured to be −151.9(9)° and −171.8(1)°, respectively. Therefore, conformer A adopted an anti conformation ( Supplementary Fig. 9a ) and conformer B adopted an unusual high -anti conformation with the almost eclipsing of O4B′-C1B′ and N8B-C7B bonds ( Supplementary Fig. 9b ). The high -anti conformation was very scarce for other nucleosides except for azanucleosides and formycin [45] . In the current case, B conformer appeared to be stabilized through an unprecedently reported intermolecular H-bond between 2′-OH and N1 of base moiety as mentioned above ( Fig. 3b ). 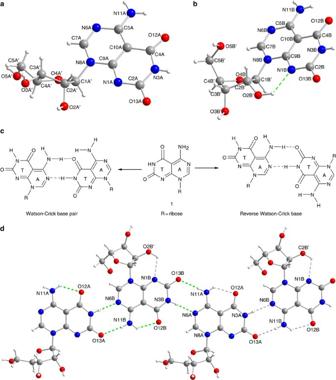Figure 3: Structures of two monomeric conformers and the base pair motifs between them. (a) Conformer A adopts ananticonformation with an N-type (3′-endo) sugar puckering and 5′-OH atapposition. (b) Conformer B adopts high-anticonformation with an S-type (3′-exo) sugar puckering and 5′-OH atscposition. The intramolecular H-bond between 2′-OH and N1B is shown in green colour. (c) Two possible base pair motifs of compound1. (d) A detailed view of the reverse Watson–Crick base pairs in the solid state of1. The repeated hydrogen bonds unit connecting conformers A and B together in the whole assembly is highlighted in green colour. Atoms are coded as follows: red, oxygen; blue, nitrogen; gray, carbon; white, hydrogen. Figure 3: Structures of two monomeric conformers and the base pair motifs between them. ( a ) Conformer A adopts an anti conformation with an N-type (3′- endo ) sugar puckering and 5′-OH at ap position. ( b ) Conformer B adopts high- anti conformation with an S-type (3′- exo ) sugar puckering and 5′-OH at sc position. The intramolecular H-bond between 2′-OH and N1B is shown in green colour. ( c ) Two possible base pair motifs of compound 1 . ( d ) A detailed view of the reverse Watson–Crick base pairs in the solid state of 1 . The repeated hydrogen bonds unit connecting conformers A and B together in the whole assembly is highlighted in green colour. Atoms are coded as follows: red, oxygen; blue, nitrogen; gray, carbon; white, hydrogen. Full size image Sugar puckering (defined by pseudorotation phase angle, P) is the driving force to dominate the whole conformations of nucleosides and even of DNA/RNA. Among two principal puckering modes (C3′- endo , North or C2′- endo , South), ribonucleosides invariably adopt C3′- endo (North) puckering. Here, we found, conformer A adopted a typical N-type conformation with a twist of C3′- endo ( 3 T 4 , P =20.7(2)°, τ m =34.1(7)°), but conformer B adopted an S-type conformation with a twist of C3′- exo ( 3 T 4 , P = 206.0(3)°, τ m =32.5(5)°), which resulted from the unusual intramolecular H-bond between 2′-OH and N1 mentioned above. The orientation of the 5′-hydroxyl group relative to the furanose, defined by the torsion angle γ (O5′–C5′–C4′–O4′), is also a crucial structural parameter. Conformer A was in ap ( gauche , trans ) range with the O5A′-OH at equatorial position and pointing into the sugar ring ( γ =68.6(5)°). Conformer B was in + sc ( gauche , gauche ) range with the O5B′-OH at axial position and pointing outside the sugar ring ( γ =−69.1(3)°). Consequently, the distance between 5′-OH and 3′-OH of conformer B is more stretched than that for conformer A ( Fig. 3a,b ). For the normal bidentate adenine–thymine base pairs, not only Watson–Crick but also reverse Watson–Crick pattern is possible, and the latter will lead to the formation of a parallel-stranded duplex DNA [46] , [47] . The current J-AT system is endowed with the same options ( Fig. 3c ), but only the reverse Watson–Crick base pairs were found in the single crystal ( Fig. 3d ). Strikingly, these base pairs existed invariably between conformers A and B through the faces of adenine and thymine ( Fig. 3d , N3B-H3B—N6A, N11A-H11A—O13B, N3A-H3A—N6B, N11B-H11B—O13A), which extended to form a linear ribbon structure with an alternating arrangement of conformers A and B with ribose residues located on both the sides. In addition, an intramolecular hydrogen bond between N11-H and O12 was found in both conformers, which was a general characteristic for the J-AT system. At the 3D supramolecular level, a novel multilayered structure with complicated hydrogen bond networks was formed ( Fig. 4a–d ). The layers can be clearly seen from Fig. 4a , but adjacent base pair layers are not stacked ( Fig. 4b and Supplementary Fig. 10 ). To display the complexity clearly, here we present the whole hydrogen bond interactions in three categories: A–A, B–B and A–B interactions across different layers with the participation of some water molecules. The A–A conformer interactions are displayed in Fig. 4c : one water molecule links together three A conformers from three neighboring layers with four hydrogen bonds and a direct intermolecular hydrogen bond of O5A′–H5A′–O13A tethers the sugar residue and base moiety of two A conformers from adjacent layers together. The B–B conformer interactions are displayed in Fig. 4d : one water molecule acts as a bridge joining two B-conformers from the upper and lower layers with bifurcated hydrogen bonds and a direct intermolecular hydrogen bond of C1B′-H1B′—O13B connects the sugar residue and base moiety of two B conformers between the middle and the lower layer. The interactions of conformers A–B are more complicated and can be seen from Fig. 4b : The 3′-OH of one conformer A is connected to the 2′-OH of one conformer B at the same layer through a water molecule. The 2′-OH of one conformer A is directly connected to the 2′-OH of one conformer B (O2A′–H2A′–O2B′). Another water molecule (O15) holds two conformers A and one conformer B together. There is another direct hydrogen bond holding conformers A and B together from the adjacent layers (O3A′–H3A′–O3B′, N11A–HA–O5B′). Totally, there are nine intermolecular hydrogen bonds acting as the repeating unit connecting conformer A and B together. 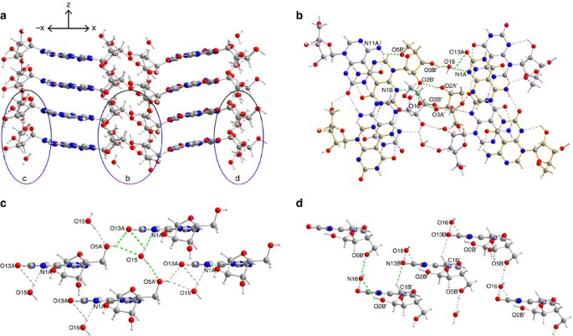Figure 4: Complicated hydrogen bond networks of compound1. (a) The overall multilayered supramolecular structure of compound1. (b) The interactions between conformers A and B (viewed throughzdirection ofa). The base moieties of adjacent layers are not stacked and the covalent bonds of different layers are displayed in yellow or purple colour, respectively. (c) The interactions between conformer A and A (viewed through −xdirection ofa). (d) The interactions between conformer B and B (viewed throughxdirection ofa). The total repeated 20 hydrogen bonds unit crossing different layers of the whole assembly is highlighted in green colour. Atoms are coded as follows: red, oxygen; blue, nitrogen; gray, carbon; white, hydrogen. Figure 4: Complicated hydrogen bond networks of compound 1 . ( a ) The overall multilayered supramolecular structure of compound 1 . ( b ) The interactions between conformers A and B (viewed through z direction of a ). The base moieties of adjacent layers are not stacked and the covalent bonds of different layers are displayed in yellow or purple colour, respectively. ( c ) The interactions between conformer A and A (viewed through − x direction of a ). ( d ) The interactions between conformer B and B (viewed through x direction of a ). The total repeated 20 hydrogen bonds unit crossing different layers of the whole assembly is highlighted in green colour. Atoms are coded as follows: red, oxygen; blue, nitrogen; gray, carbon; white, hydrogen. Full size image Therefore, for compound 1 , a very complicated hydrogen bond network (20 hydrogen bonds in total from both base and sugar parts) is repeated infinitely in the whole assembly to form the 3D multilayered supramolecular structure in single-crystal state. Obviously, both base moieties and the sugar residues are intrinsic deterministic factors (through proper conformation) to direct the three-dimensional superstructure shape. Meanwhile, the dried flower-shaped powders obtained from the SEM samples were also analysed by XRPD [48] . The pattern of XRPD displayed close similarity with the pattern simulated from the single-crystal data ( Supplementary Fig. 11 ), suggesting that the flower-shaped solution aggregate on fast cooling adopted the same interactions. The phenomenon that compound 2 (lacking the 2′-OH group compared with compound 1 ) could only form the microsphere suggested that the 2′-OH group might play a key role in this anisotropic growth process. Its importance was also revealed here by the multiple participations in the whole H-bond network. To further confirm this suppose, we designed and synthesized the 5′-deoxyrbonucleoside ( 3 ) and 3′-deoxyribonucleoside ( 4 ); both conserved the 2′-OH group but one -OH group was removed like the case of 2 , to see whether or not they could still form the flower-shaped superstructure in solution state. Construction of flower-shaped superstructures 5′-Deoxyribonucleoside ( 3 ) was synthesized from the sugar donor of 1, 2, 3- tri - O -acetyl-5-deoxy- β - D -ribofuranose. The initial attempts to synthesize 3′-deoxyribonucleoside ( 4 ) through selective deoxygenation of 1 failed due to the poor solubility of free J-AT nucleoside in various organic solvents. Consequently, 4 was obtained via Vorbrueggen glycosylation procedures with SnCl 4 as the catalyst and 1,2- di - O -acetyl-5- O -benzoyl-3-deoxy- β - D -ribofuranose as the sugar donor ( Supplementary Figs 12–17 ). As we anticipated, both compound 3 and 4 can form flower-shaped superstructures, which confirmed the key role of the 2′-OH group: once it exists in the molecule, the flower shape retains. Of course, the different molecular structures also led to different overall shapes of the ‘flowers’: spiral form for 3 and ball flower for 4 , but both retained the ‘petals’ as shown in Fig. 5 . Fortunately, the single crystal of 4 was obtained in aqueous solution by a slowly cooling procedure ( Supplementary Data 2 ). The differences of inner workings between 1 and 4 can be seen clearly in the single-crystal state. There were also two conformers ( anti and high -anti ) for compound 4 in equal amounts, which were connected together by the reverse Watson–Crick base pairs ( Supplementary Figs 18,19 ) as well. However, owing to lack of the 3′-OH group, the sugar puckering of both conformers of 4 adopted N-type modes without the intramolecular hydrogen bond of 2′-OH-N1. Instead, the high -anti conformation of conformer B was locked through the intermolecular hydrogen bonds with the participation of 2′-OH, in the context of the whole assembly. In general, the whole supramolecular assembly was formed by spatial repeating of 13 hydrogen bonds involving both base and sugar parts ( Fig. 5c , Supplementary Fig. 20 ). The four hydrogen bonds formed around 2′-OH (O2A′–H2A′–O5B′, O2A′–N11A–H11A, O2B′–H2B′–O5A′, O2B′–N11B–H11B) clearly indicated its key roles in directing the whole assembly. It is worth mentioning that water molecules were totally expelled from the whole assembly of 4 . These differences might suggest that the flower formed by 4 was more compact than 1 . 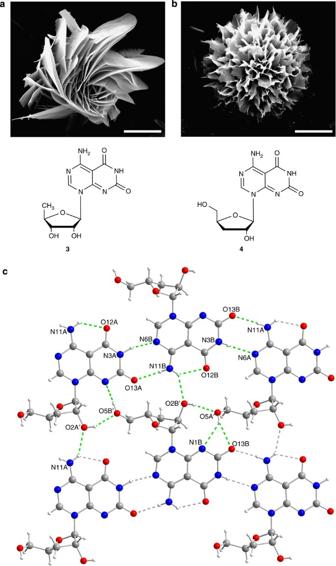Figure 5: SEM images of compounds 3–4 and the single-crystal structure of compound4. (a) Spiral flower-shaped superstructure formed by3in water (0.2 mg ml−1). (b) Ball flower-shaped superstructure formed by4in water (0.2 mg ml−1). (c) The single-crystal structure of4. The repeated unit of 13 intra and intermolecular hydrogen bonds is highlighted in green colour. Atoms are coded as follows: red, oxygen; blue, nitrogen; gray, carbon; white, hydrogen. Scale bars, (a,b) 10 μm. Figure 5: SEM images of compounds 3–4 and the single-crystal structure of compound 4 . ( a ) Spiral flower-shaped superstructure formed by 3 in water (0.2 mg ml −1 ). ( b ) Ball flower-shaped superstructure formed by 4 in water (0.2 mg ml −1 ). ( c ) The single-crystal structure of 4 . The repeated unit of 13 intra and intermolecular hydrogen bonds is highlighted in green colour. Atoms are coded as follows: red, oxygen; blue, nitrogen; gray, carbon; white, hydrogen. Scale bars, ( a , b ) 10 μm. Full size image Molecular recognition by compound 1 The base moiety of J-AT nucleoside derivatives has one face of adenine H-bond array and the other face of thymine array. In addition to the self-complementarity, J-AT, in principle, can be competitively base paired with either adenosine or uridine/thymidine. The influences of the complementary or non-complementary natural ribonucleosides on supramolecular shapes were investigated by adding them into the aqueous solution of 1 (0.2 mg ml −1 ) and comparing the new structures with the corresponding structures of individual normal nucleosides ( Supplementary Fig. 21 ). Initially, we supposed that both adenosine and uridine could interrupt the microflower formation of 1 because the elongation of the linear ribbon structure will be terminated by J-AT-A or J-AT-U base pairs. Indeed, the flower-shaped structure of 1 completely disappeared in the case of J-AT+A (1:1) mixture, with the formation of microspheres ( Fig. 6a ), which was completely different from either the J-AT microflower or the adenosine’s fiber-shaped structure. This meant the J-AT and adenosine were indeed hybridized. Contrary to our anticipation, compound 1 did not pair with uridine easily. When 1 equiv. U was added, the microflower remained intact ( Fig. 6b ). When 5 equiv. U was added, an amazing chimerical structure with ‘petals’ protruding from the smooth membrane formed by uridine was observed. This chimerical morphology indicated the partial base pairs between 1 and uridine ( Fig. 6c ). The different base pair properties between 1 and adenosine or uridine can be explained by the rotation barrier of the glycosyl bond ( Supplementary Fig. 22 ). Current results suggested the anti conformation was predominant in solution as well, which is consistent with the single-crystal structures ( anti and high -anti conformers). 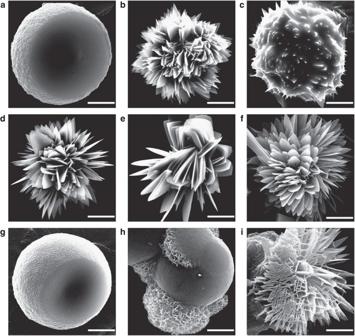Figure 6: Chimeric morphologies formed by mixing J-AT with other nucleosides. (a) J-AT:Adenosine (1:1 mole ratio). (b) J-AT:Uridine (1:1 mole ratio). (c) J-AT:Uridine (1:5 mole ratio). (d) J-AT:Cytidine (1:1 mole ratio). (e) J-AT:Cytidine (1:5 mole ratio). (f) J-AT:Guanosine (1:1 mole ratio). (g) J-AT:Guanosine (1:5 mole ratio). (h) J-AT:compound2(1:1 mole ratio). (i) J-AT:J-TA (1:1 mole ratio). Scale bars, (a,g–i), 5 μm; (b–f), 10 μm. Figure 6: Chimeric morphologies formed by mixing J-AT with other nucleosides. ( a ) J-AT:Adenosine (1:1 mole ratio). ( b ) J-AT:Uridine (1:1 mole ratio). ( c ) J-AT:Uridine (1:5 mole ratio). ( d ) J-AT:Cytidine (1:1 mole ratio). ( e ) J-AT:Cytidine (1:5 mole ratio). ( f ) J-AT:Guanosine (1:1 mole ratio). ( g ) J-AT:Guanosine (1:5 mole ratio). ( h ) J-AT:compound 2 (1:1 mole ratio). ( i ) J-AT:J-TA (1:1 mole ratio). Scale bars, ( a , g – i ), 5 μm; ( b – f ), 10 μm. Full size image 1 or 5 equiv. of cytidine was not able to interrupt the flower-shaped superstructure of 1 , in accordance with that cytosine pairs with neither the adenine face nor the thymine face of J-AT under such conditions ( Fig. 6d,e ). In addition, this result supported that the base pairs were the main force in bringing the molecules together; otherwise the cytidine could be incorporated if the interactions between riboses were the main forces. Guanosine showed a moderate influence on the microflower superstructure. The addition of 1 equiv. of guanosine did not change the overall shape of the microflower ( Fig. 6f ) with the co-existence of a tape-shaped structure from guanosine itself. By further increasing guanosine up to 5 equiv., the flower disappeared and transformed to a microsphere like in the case of adding adenosine ( Fig. 6g ). This phenomenon was practically in accordance with the well-documented G-A and G-T/G-U mismatches due to the guanine’s multiple hydrogen-bonding sites. Next, the effect of incorporating J-AT analogues with different sugar residues was also investigated. The SEM experiments showed that chimerical supramolecular structures consisted of microflowers and microspheres were formed in the mixed solution containing equal amounts of compounds 1 and 2 ( Fig. 6h ). Another chimerical structure combining microflowers with interwoven nanobundles was also observed in the mixed solution containing equal amounts of 1 and J-TA nucleoside; the latter formed nanobundles by itself ( Fig. 6i , Supplementary Fig. 23 ). Therefore, the specific molecular recognition property of J-AT nucleoside was retained, indicated by the different hybridized shapes, which is beneficial for further functionalizing of this structure through specific non-covalent interactions. Previously, during our research of some Janus-type nucleoside analogues concerning their antiviral and antitumor activities, in parallel we found that compound 1 could form a beautiful flower-shaped superstructure in different solutions. However, there was no thorough insight into the dynamic formation process and the molecular architecture of this special nucleoside self-assembly with high resolution at that time. Considering the scientific and practical significance of complex natural mimic-shaped chemical structures, we intended to investigate this flower-shaped nucleoside superstructure thoroughly, including its formation mechanism, the inner interactions at the atomic level, and how the modified structures and its molecular recognition properties influence the superstructures. In general, the experimental results from DLS, NMR and SEM suggested a two-staged mechanism (from microsphere to a complete flower-shaped state) for the anisotropic growth of the flower-shaped superstructure. In addition, the DSC provided the thermodynamic parameters for such biphasic process. Therefore, to form such complex morphology, first the non-specific H-bonds hold fast the individual molecules together to form the nucleation and grow into a microsphere, and then once they are held closer a reorganizing process follows. In order to form specific base pairs, the correct conformation around the glycosyl bond was required (high -anti conformation in this case), which further influenced the sugar puckering. Consequently, all the hydroxyl groups were rearranged again in a fixed spatial direction to form an energy-favourable complicated H-bond network, which led to the fine tuning of the whole system into a branched flower-shaped superstructure. The atomic-level interactions of the single crystal consisting of complicated hydrogen bond-mediated networks have been revealed by X-ray analysis, which was very rarely reported for related topics [45] . This information was fundamental to understanding all the forces and connectivities of such complicated superstructures. An added value is that this structure is a nice example of a H-bonded system in aqueous environment, which is rather difficult to form due to the competition of water molecules [49] , [50] . We also carried out XRPD experiments, which bridged the structures between the powders prepared from the flower-shaped solution state and that prepared from the single-crystal state by comparing the experimental pattern with the calculated pattern. The results suggested the flower-shaped solution aggregate on fast cooling adopted the same interactions as the single-crystal state. The reproduction of similar flower-shaped morphologies by related compounds 3 and 4 by modifying the hydroxyl groups proved the viabilities of using this new type of compounds to build complex superstructures with their unique inner working and meanwhile confirmed our doubts about the relationship between the single molecular structural parameter and the shapes of the final supramolecular assemblies. This information is also very helpful for us to construct or functionalize such complex-shaped structure in the future. The most powerful property of nucleosides is their unique base pair recognition, which is the base of DNA/RNA replications and transcriptions [29] , [30] . These recognition properties were also employed in the current case to build rather interesting hybrid morphologies, which might expand its usages greatly. In summary, the two-staged formation process of a complicated flower-shaped supramolecular structure was revealed by various techniques. The sophisticated hydrogen bond networks have been revealed by X-ray analysis. Such complex-shaped superstructures can be constructed and expanded to related chemical entities by modifying certain functional groups as well. Therefore, nucleosides can also play an important role, with the combination of the rich chemistry of both heterocycles and sugars and its 3D conformational flexibility, to fabricate more complex chemical architectures in the supramolecular self-assembly area. General All chemicals were commercially available. The solvents and reagents were analytic pure. Solvents 1,2-dichloroethane and acetonitrile were purified by distilling from P 2 O 5 . Thin-layer chromatography (TLC) was performed on an aluminium sheet covered with silica gel 60 F254 (0.2 mm, Merck, Germany). Flash column chromatography (FC) was carried out with silica gel 60 (Haiyang chemical company, PR China) at 0.4 bar. NMR spectra were recorded on a AV II (Bruker, Germany) spectrometer at 400 and 600 MHz; the δ values in p.p.m. are relative to Me 4 Si as internal standard; High-resolution mass spectra were measured with a mass analyser (Q-TOF, Bruker, Germany). The UV absorption spectra were recorded on a DU-800 spectrophotometer (Beckman, US), λ max in nm, ε in dm 3 mol −1 cm −1 ; the XRPD spectra were measured on X'Pert Pro MPD. The DLS spectra were recorded on JL-6000 and Nano-ZS (Malvern); differential scanning calorimetry (DSC) measurements were carried out using a VP-DSC microcalorimeter (Microcal, Northampton, MA). SEM experiments SEM was performed using a high-resolution INSPECT F50. All SEM images were obtained without staining. Samples were prepared by dissolving corresponding compounds in H 2 O (0.2 mg ml −1 ). The solutions were heated to 100 °C and allowed to cool to room temperature. The samples were taken for SEM experiments at specified time intervals. For the time-elapsing experiments, 100 μl sample solution was taken at different time intervals (0, 20, 40 min, 1, 2, 3, 5, 8, 10, 12, 14, 16, 18, 20, 22 and 24 h) to be observed under SEM. DSC experiments Microcalorimetry experiments were performed on VP-DSC microcalorimeter driven by a DSC-run software. Compound 1 was dissolved at a concentration of 0.4 mg ml −1 in water. Solutions were carefully degassed prior to their utilization and their thermal profiles were analysed in the 25–80 °C temperature range at a scan rate of 0.5 °C min −1 . Synthetic procedures All compounds were synthesized from commercially available materials and characterized by 1 H, 13 C NMR spectroscopy and HRMS. Crystallographic study of 1 and 4 Single crystals were obtained by slowly cooling the corresponding saturated solution in steps of 0.5 °C h −1 from 100 to 30 °C. Proper-sized single crystals of compounds 1 and 4 were stabilized into a tiny glass tube including mother liquor with epoxy resin to minimize solvent loss. Crystal data were collected on Bruker Apex II. Synthesis of Compound 9 Compound 5 (5-aminopyrimido[4,5-d]pyrimidine-2,4(1H,3H)-dione) [51] (500 mg, 2.79 mmol) was suspended in hexamethyldisilazane (HMDS, 50 ml). After the mixture being stirred at 140 °C for 3 min, trimethylsilyl chloride (TMSCl, 500 μl) was added. The mixture was stirred under refluxing for about 10 h until it turned clear. Then, the solution was evaporated to remove excess HMDS and the silylated base 6 was obtained and immediately used without further purification. At room temperature, to this silylated base residue was added 1,2-dichloroethane:acetonitrile (1:1, 50 ml) followed by adding 1,2,3,- tri - O -acetyl-5-deoxy- β - D -ribofuranose ( 7 ). This mixture was cooled to 0 °C and SnCl 4 (500 μl) was added as catalyst. After the mist vanished, the reaction was brought to room temperature and the stirring was continued for 1 h. Then, saturated NaHCO 3 aqueous solution (20 ml) was added at 0 °C to quench the reaction. Next, 30 ml CH 2 Cl 2 was added. The organic phase was collected and dried with anhydrous Na 2 SO 4 . After the evaporation of the CH 2 Cl 2 , the residue was applied to FC (CH 2 Cl 2 :methanol=99:1) and compound 9 (550 mg, 52%) was obtained as colourless powder. TLC (CH 2 Cl 2 :MeOH, 99:1 v/v): R f =0.2; UV/Vis: λ max (MeOH)/nm ( ε /dm 3 mol −1 cm −1 ): 232 (29,355), 250 (54,418), 276 (14,913), 273 (4,798); 1 H NMR(400 MHz, DMSO- d 6 ): δ 1.40 (d, J =4.00 Hz, 3H, 5′-CH 3 ), 2.07 (d, J =8.80 Hz, 6H, OAc), 4.19 ( t , J =4.4 Hz, 1H, 4′-H), 5.29 ( t , J =4.40 Hz, 1H, 3′-H), 5.64 (q, J =2.80 Hz, 1H, 2′-H), 6.22 (d, J =2.8 Hz, 1H, 1′-H), 8.56 (s, 1H, 7-CH), 9.09 (dd, J =2.40 Hz, J =2.00 Hz, NH 2 ), 10.83 (s, 1H, NH); 13 C NMR (100 MHz, DMSO- d 6 ): δ 18.32, 20.74, 20.81, 73.53, 74.09, 78.57, 87.34, 90.21, 152.80, 156.73, 157.73, 161.90, 165.31, 169.90, 169.93; HRMS (ESI+) m/z : calcd for: [C 15 H 17 N 5 O 7 +Na] + : 402.1026; found: 402.1028. Synthesis of Compound 3 Compound 9 (200 mg, 0.52 mmol) was suspended in freshly prepared 15 ml 0.10 M sodium methoxide. The reaction mixture was stirred at r.t. for 20 min. After neutralization with diluted acetic acid, the mixture was filtrated and the residue was washed with MeOH and H 2 O three times to get the product 3 (140 mg, 91%); UV/Vis: λ max (MeOH)/nm ( ε /dm 3 mol −1 cm −1 ): 233 (16,787), 250 (17,520), 276 (4,833), 273 (4,798); 1 H NMR(400 MHz, DMSO- d 6 ): δ 1.33 (d, J =4.00 Hz, 3H, 5′-CH 3 ), 3.82 (t, J =3.60 Hz, 1H, 4′-H), 3.95-3.99 (m, J =4.00 Hz, 3′-H), 4.23 (t, J =2.80 Hz, 2′-H), 5.13 (s, 1H, 3′-OH), 5.52 (s, 1H, 2′-OH), 6.13 (d, J =2.40 Hz, 1H, 1′-H), 8.40 (s, 1H, 7-CH), 9.02 (s, 2H, NH 2 ), 10.81 (s, 1H, NH); 13 C NMR (100 MHz, DMSO- d 6 ): δ 18.63, 74.33, 74.62, 80.17, 87.43, 90.70, 151.86, 156.95, 158.21, 161.94, 165.43; HRMS (ESI-) m/z : calcd for: [C 11 H 13 N 5 O 5 -H] − : 294.0838; found: 294.0837. Synthesis of Compound 10 Compound 5 (1.00 g, 5.60 mmol) was suspended in hexamethyldisilazane (HMDS) (50 ml) and stirred at 140 °C for about 3 min; then trimethylsilyl chloride (TMSCl, 1 ml) was added. The reaction was stirred at reflux until the mixture became clear. Next, the solution was evaporated to remove HMDS. The silylated base 6 was obtained, which was immediately used in the next step without further purification. Dry 1,2-dichloroethane (45 ml) was added to the pot containing silylated base 6 and stirred. 1,2- di - O -acetyl-5- O -benzoyl-3-deoxy- β - D -ribofuranose 8 (920 mg, 2.90 mmol) dissolved in dry acetonitrile (45 ml) was added to the above solution. SnCl 4 (952 μl) was added as catalyst at 0 °C. After the mist vanished, the reaction mixture was stirred at room temperature for about 2 h, and saturated NaHCO 3 aqueous solution (60 ml) was added at 0 °C to quench the reaction; CH 2 Cl 2 (3 × 60 ml) was used to extract the organic phase. After drying with anhydrous Na 2 SO 4 , the organic phase was evaporated. The residue was applied to FC (CH 2 Cl 2 : methanol=98:2) and afforded compound 10 (50%, 1.23 g). TLC (CH 2 Cl 2 :MeOH, 98:2 v/v): R f =0.2; UV/Vis: λ max (MeOH)/nm ( ε /dm 3 mol −1 cm −1 ): 231 (21,016), 251 (25,376), 277 (6,515); 1 H NMR (600 MHz, DMSO- d 6 ): δ 2.15 (s, 3H, CH 3 ), 3.35 (s, 2H, 3′-H), 4.10 (d, J =3.40 Hz, 1H,4′-H), 4.63–4.80 (m, 3H, 2′-H and 5′-H), 6.37 (s, 1H, 1′-H), 7.53-8.03 (m, 5H, H-Ar), 8.43 (s, 1H, C7H), 9.01 (d, J =7.50 Hz, 2H, NH 2 ), 10.82 (s, 1H, NH). 13 C NMR (150 MHz, DMSO- d 6 ): δ 21.14, 55.38, 58.09, 62.77, 78.23, 81.49, 82.22, 87.36, 89.53, 129.28, 129.76, 134.03, 151.06, 156.83, 157.86, 161.86, 165.34, 166.02, 169.77; HRMS (ESI+) m/z : calcd for [C 20 H 19 N 5 O 7 +Na] + : 464.1182; found 464.1177. Synthesis of Compound 4 Compound 9 (100 mg, 0.23 mmol) was dissolved in 0.5 M NaOMe/MeOH (7 ml), and the solution was refluxed at 75 °C for about 10 min. After cooling to room temperature, the solution was neutralized with diluted acetic acid to pH 6.5 and precipitate was formed. After filtration the precipitate was washed with methanol (3 × 2 ml) and water (1 × 2 ml). Target compound 4 was obtained as a white powder by vacuum drying (50 mg, 74%). UV/Vis: λ max (MeOH)/nm ( ε /dm 3 mol −1 cm −1 ): 233 (14,294), 250 (25,260), 276 (5,787); 1 H NMR (600 MHz, DMSO- d 6 ): δ 1.71-1.74 (m, 1H, 3′-H), 2.03-2.08 (m, 1H, 3′-H), 3.60 (d, J =12.50 Hz, 1H,5′-H), 3.87-3.90 (m, 1H, 5′-H), 4.34 (s, 1H, 4′-H), 4.40-4.47 (m, 1H, 2′-H), 5.31 (t, J =4.70 Hz, 1H, 5′-OH), 5.63 (d, J =3.80 Hz, 1H, 2′-OH), 6.04 (s, 1H, 1′-H), 8.86 (s, 1H, NH), 8.92 (s, 1H, NH), 8.96 (s, 1H, CH), 10.77 (s, 1H, NH). 13 C NMR (150 MHz, DMSO- d 6 ): δ 32.56, 61.04, 75.76, 82.65, 87.55, 93.13, 151.40, 157.05, 158.08, 162.13, 165.45; HRMS (ESI+) m/z : calcd for [C 11 H 13 N 5 O 5 +Na] + : 318.0815; found 318.0809. Accession codes: The X-ray crystallographic coordinates for structures reported in this Article have been deposited at the Cambridge Crystallographic Data Centre (CCDC), under deposition number CCDC: 940972 ( 1 ) and 946631 ( 4 ). These data can be obtained free of charge from The Cambridge Crystallographic Data Centre via www.ccdc.cam.ac.uk/data_request/cif . How to cite this article: Zhao, H. et al. Complex self-assembly of pyrimido[4,5- d ]pyrimidine nucleoside supramolecular structures. Nat. Commun. 5:3108 doi: 10.1038/ncomms4108 (2014).